Crystal structure of the human thioredoxin reductase–thioredoxin complex Thioredoxin reductase 1 (TrxR1) is a homodimeric flavoprotein crucially involved in the regulation of cellular redox homeostasis, growth, and differentiation. Its importance in various diseases makes TrxR1 a highly interesting drug target. Here we present the first crystal structures of human TrxR1 in complex with its substrate thioredoxin (Trx). The carboxy-terminal redox centre is found about 20 Å apart from the amino-terminal redox centre, with no major conformational changes in TrxR or Trx. Thus, our structure confirms that the enzyme uses a flexible C-terminal arm for electron transport to its substrates, which is stabilized by a guiding bar for controlled transfer. This notion is supported by mutational analyses. Furthermore, essential residues of the interface region were characterized both structurally and functionally. The structure provides templates for future drug design, and contributes to our understanding of redox regulatory processes in mammals. The intracellular redox milieu is supported by the thioredoxin system, composed of the flavoenzyme thioredoxin reductase (TrxR, EC 1.8.1.9), NADPH, and its main substrate thioredoxin (Trx). TrxR reduces the disulphide of Trx using NADPH as the source of reducing equivalents. During catalysis, the electrons are transferred from NADPH to FAD, then to the buried amino-terminal active site, to the carboxy-terminal active site of the other TrxR subunit, and from there to the substrate at the protein's surface. TrxR influences essential cellular processes either indirectly through reduced thioredoxin or directly by reducing substrates acting in DNA and selenium metabolism, antioxidant defence, or cell growth regulation and apoptosis [1] . The central and diverse functions of the thioredoxin system currently make it one of the most attractive targets for antitumour drug development [2] , [3] . In mammals, three types of TrxRs have been characterized: the cytosolic form TrxR1 (also known as TR1 or TXNRD1) [4] , the mitochondrial form TrxR2 (also known as TR3 or TXNRD2) [5] , [6] , and thioredoxin glutathione reductase (TGR, also known as TrxR3, TR2 or TXNRD3) that occurs in the microsomal fraction of testis tissue [7] . The hybrid enzyme TGR possesses an N-terminal glutaredoxin-domain in addition to a C-terminal selenocysteine-containing redox centre and therefore combines TrxR and GR (glutathione reductase) activities [7] . Furthermore, mammalian cells contain two ubiquitously expressed Trxs [1] , [8] . Trx1 is a cytosolic and nuclear protein, whereas Trx2 is targeted to mitochondria [1] , [8] . Cytosolic Trx1 was the major substrate captured by immobilized TrxR1, indicating that the main function of TrxR1 is to reduce Trx1 [9] . TrxRs belong to a family of homodimeric pyridine nucleotide disulphide oxidoreductases with high homology to GRs. The overall fold of human TrxR1 resembles other homodimeric pyridine nucleotide disulphide oxidoreductases such as rat TrxR1 (ref. 10 ) and human GR [11] , [12] . Each subunit contains a binding domain for FAD and NADPH, an interface domain, and a discrete active centre [10] , [13] . Human TrxR1 and GR share a high active site residue similarity at the cofactor and substrate binding sites as well as a similar reaction mechanism with respect to the reductive half-reaction [10] . The structural and functional characteristics of GR have been studied for many years, and detailed information on the mechanism is available [12] . However, much less is known about the oxidative half-reaction of TrxRs. Mammalian TrxRs contain selenocysteine (Sec) as the penultimate amino acid, which is important for high catalytic efficiency [14] . The species-specific usage of the selenocysteine insertion sequence element makes a heterologous expression of the mammalian enzyme difficult—a challenge which has been tackled by different groups. Recently, Cheng et al . [15] solved two crystal structures of selenocysteine containing rat TrxR1 (rTrxR1), one with an oxidized and the other one with a reduced C-terminal active site. The overall structures are similar to other previously published crystal structures of mutated TrxR1, where the selenium-atom is replaced by a sulphur atom [10] , [13] , [16] (Debreczeni JE et al ., unpublished result. PDB code 2cfy). In the rTrxR1 structure with the oxidized C-terminal active site, the selenenyl–sulphide motif is found near the side chain of Tyr116 (PDB code 3eao) [15] . This course of the C-terminal arm is similar to the conformation in subunit E of the crystal structure of a U498C mutant of hTrxR1 (PDB code 2j3n) [16] , which also contains the disulphide motif near the side chain of Tyr-116. The similar conformation of the oxidized C-terminal arm in the hTrxR1 U498C mutant as well as in the Sec-containing rTrxR1 wild-type structure indicate that the hTrxR1 U498C mutant can be used to study mechanistic details. Using double mutants of hTrxR1 C497S,U498C and hTrx1 C35S,C73S , we trapped the intermediate state of the oxidative half-reaction. We obtained crystals from this mutant protein complex and solved the three-dimensional structure by X-ray analysis at a resolution down to 2.2 Å. Our observed complex structure differs fundamentally from all previously published models of the hTrxR1–hTrx1 complex and provides new insights into the catalytic mechanism of large, eukaryotic TrxRs. Generation and purification of the hTrxR1–hTrx1 complex To catch human TrxR1 in an intermediate state where its substrate thioredoxin is bound, a stabilization of the complex is required. Therefore, we created three C-terminal active site mutants of hTrxR1 (hTrxR1 C497S,U498C , hTrxR1 U498S , and hTrxR1 C497_trunc ) and tested them against three mutants of hTrx1 (hTrx1 C73S , hTrx1 C32S,C73S , and hTrx1 C35S,C73S ; Methods section). For complex formation we incubated the hTrxR1 mutants with NADPH and the respective hTrx1 mutants. Under the conditions tested, only hTrxR1 C497S,U498C and hTrx1 C35S,C73S were able to form a complex that could be isolated by gel filtration chromatography and was stable in non-reducing SDS–PAGE ( Fig. 1 ). This protein sample yielded crystals of the hTrxR1–hTrx1 complex that could be analysed by X-ray crystallography. 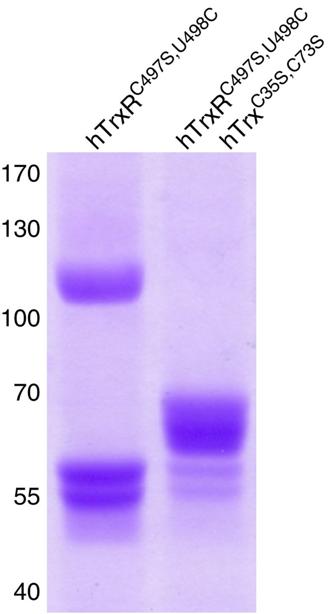Figure 1: hTrxR1C497S,U498Cforms a stable complex with hTrx1C35S,C73S. Coomassie staining of a non-reducing 4–12% SDS–PAGE gel. The left lane shows hTrxR1C497S,U498Cwithout hTrx1C35S,C73Sbound to it. The band∼114 kDa corresponds to the dimer, the band∼57 kDa to the monomer of hTrxR1C497S,U498C. The right lane shows the complex between hTrxR1C497S,U498Cand hTrx1C35S,C73S. The pronounced band∼67 kDa belongs to a monomer band of hTrxR1C497S,U498Cwith one molecule of hTrx1C35S,C73Sbound to it. The lower and weaker bands around∼57 kDa of this non-reducing gel belong to hTrxR1C497S,U498C, where hTrx1C35S,C73Shas been cleaved off due to heating of the sample. The amount of free, uncomplexed hTrxR1C497S,U498Cgrew with increasing incubation time at 95 °C before sample loading (data not shown). Conformational changes and changes in interacting forces, especially in the C-terminal region of hTrxR1 upon binding of hTrx1 are most likely the reason for the absence of a TrxR-homodimer band in this non-reducing SDS gel. Figure 1: hTrxR1 C497S,U498C forms a stable complex with hTrx1 C35S,C73S . Coomassie staining of a non-reducing 4–12% SDS–PAGE gel. The left lane shows hTrxR1 C497S,U498C without hTrx1 C35S,C73S bound to it. The band ∼ 114 kDa corresponds to the dimer, the band ∼ 57 kDa to the monomer of hTrxR1 C497S,U498C . The right lane shows the complex between hTrxR1 C497S,U498C and hTrx1 C35S,C73S . The pronounced band ∼ 67 kDa belongs to a monomer band of hTrxR1 C497S,U498C with one molecule of hTrx1 C35S,C73S bound to it. The lower and weaker bands around ∼ 57 kDa of this non-reducing gel belong to hTrxR1 C497S,U498C , where hTrx1 C35S,C73S has been cleaved off due to heating of the sample. The amount of free, uncomplexed hTrxR1 C497S,U498C grew with increasing incubation time at 95 °C before sample loading (data not shown). Conformational changes and changes in interacting forces, especially in the C-terminal region of hTrxR1 upon binding of hTrx1 are most likely the reason for the absence of a TrxR-homodimer band in this non-reducing SDS gel. Full size image Structure determination We obtained monoclinic (space group P2 1 ) and orthorhombic crystals (space group P2 1 2 1 2 1 ) of hTrxR1 C497S,U498C in complex with its substrate hTrx1 C35S,C73S ( Table 1 ). The asymmetric unit of both crystal types contained two copies of the hTrxR1–hTrx1 complex, thereby maintaining the usual TrxR dimer. The monoclinic structure was solved at 2.6 Å resolution via the molecular replacement method, using hTrx1 (PDB code 1aiu) [17] and hTrxR1 (PDB code 2j3n) [16] as search models. Interestingly, all automatic program packages identified the correct position of the hTrxR1 dimer but failed to identify any of the hTrx1 substrates. However, the 2Fo-Fc map revealed regions of helical density that served to manually place one hTrx1 molecule. The second hTrx1 molecule was inserted into the asymmetric unit through an educated guess (Methods section) so that the two complexes in the asymmetric unit were similar. The orthorhombic structure was solved by the molecular replacement method, using the structure of the monoclinic crystals as a search model. The overall temperature factors of the structures were 52.7 (monoclinic) and 40.4 (orthorhombic) Å 2 . The structures were refined to R free =29.7% (monoclinic) and 27.7% (orthorhombic) ( Table 1 ). The monoclinic and orthorhombic structures are essentially similar—with an r.m.s. of 0.6 Å for 1,194 C α -atoms of two complexes. Differences were mainly due to crystal packing forces and due to the position of the substrate hTrx1 ( Fig. 2 ) and some loops at the surface. Except for some (5-to-8) N-terminally located residues of hTrxR1, the structures were well defined by the electron density. In particular, all cysteine residues were clearly identified with temperature factors below the overall mean. Table 1 Data collection and refinement statistics. 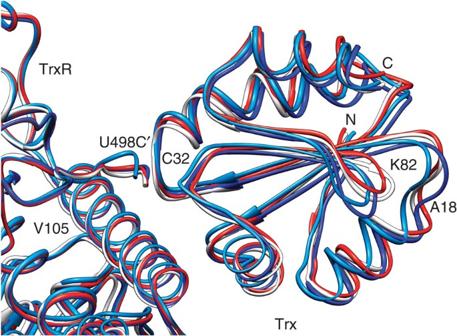Figure 2: Superimposed structures of the four hTrxR–hTrx complexes. We used a ribbon representation to show the different positions of the Trx molecules in the four complexes (orthorhombic: grey and cyan; monoclinic: blue and red). There are only slight differences around the intra-molecular disulphide between U498C′hTrxR1and C32hTrx1but for example in the regions around K82 and around A18 the distance between Cα-atoms increases up to 4 Å. Full size table Figure 2: Superimposed structures of the four hTrxR–hTrx complexes. We used a ribbon representation to show the different positions of the Trx molecules in the four complexes (orthorhombic: grey and cyan; monoclinic: blue and red). There are only slight differences around the intra-molecular disulphide between U498C′ hTrxR1 and C32 hTrx1 but for example in the regions around K82 and around A18 the distance between Cα-atoms increases up to 4 Å. Full size image Overall structure The homodimeric flavoprotein TrxR1 possesses two redox centres, both of which are required for catalysis. The N-terminally located centre (Cys59 hTrxR1 , Cys64 hTrxR1 ) is buried in the protein, whereas the second, C-terminally located centre (Cys497′ hTrxR1 , Sec498′ hTrxR1 ) is positioned on a flexible, highly accessible C-terminal arm of the other subunit (residues belonging to the other subunit are primed). As described above, we used mutants of hTrxR1 (hTrxR1 C497S,U498C ) and hTrx1 (hTrx1 C35S,C73S ) to obtain crystals of the reaction intermediate between hTrxR1 and hTrx1. Both crystal types (monoclinic and orthorhombic) contained two 1:1 hTrxR1–hTrx1 complexes in the asymmetric unit. The two hTrxR1 molecules formed a twofold dimer as previously observed ( Fig. 3 ) [10] , [13] , [16] . 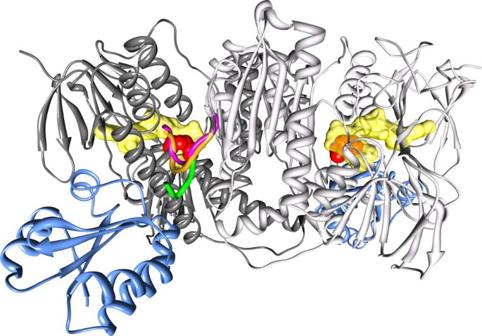Figure 3: Overview of the hTrxR1 dimer with bound hTrx1. hTrxR1 (grey) and hTrx1 (blue) are shown in ribbon representation. FAD (yellow) and the N-terminal redox centre (red) are shown in ball representation. The different conformations of the C-terminus (last 8 residues) as found in the 'oxidized waiting position', 'reduced waiting position', and in the hTrxR1–hTrx1 complex are coloured magenta, orange, and green, respectively. Molecular graphics images were produced using the UCSF Chimera package40. Figure 3: Overview of the hTrxR1 dimer with bound hTrx1. hTrxR1 (grey) and hTrx1 (blue) are shown in ribbon representation. FAD (yellow) and the N-terminal redox centre (red) are shown in ball representation. The different conformations of the C-terminus (last 8 residues) as found in the 'oxidized waiting position', 'reduced waiting position', and in the hTrxR1–hTrx1 complex are coloured magenta, orange, and green, respectively. Molecular graphics images were produced using the UCSF Chimera package [40] . Full size image As shown by our structure, complex formation of hTrxR1 with hTrx1 involves the generation of an intermolecular disulphide bond between the catalytic residues Cys32 hTrx1 and U498C′ hTrxR1 , which is supported by their neighbouring residues. The formation of the complex is further stabilized by several interactions between hTrx1 residues 58 hTrx1 to 74 hTrx1 and the helical hTrxR1 residues Glu103 hTrxR1 to Glu122 hTrxR1 ( Fig. 4 ). Owing to complex formation, Trp31 hTrx1 and Trp114 hTrxR1 are buried with their indole rings at the interface region within van der Waals distance. Trp31 hTrx1 fits into a pocket, formed by residues Ala29 hTrx1 , Met74 hTrx1 , Asn107 hTrxR1 , Gly110 hTrxR1 , Ser111 hTrxR1 , Trp114 hTrxR1 , and the mixed disulphide, whereas the indole is stacked with main chain atoms of residues 110 hTrxR1 and 111 hTrxR1 ( Fig. 5 ). Moreover, Trp31 hTrx1 forms hydrogen bonds to Asp60 hTrx1 , which forms salt bridges to Arg117 hTrxR1 in three copies of the four hTrxR1–hTrx1 complexes. The pocket residue Trp114 hTrxR1 is sandwiched between Met74 hTrx1 and Val59 hTrx1 and surrounded by residues 71 hTrx1 , 72 hTrx1 , 117 hTrxR1 , and 499′ hTrxR1 ( Fig. 4 ). 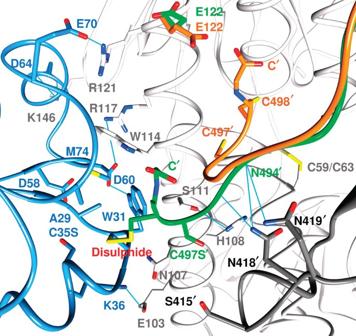Figure 4: Close-up view of the hTrxR1-hTrx1 interface. One hTrxR1 subunit is shown in light grey, the other in dark grey and the hTrx1 molecule in blue; the C-terminal arm of the complex structure is shown in green. The conformation of the C-terminal arm and of residue E122 as found in the 'reduced waiting position' are superimposed and are coloured orange. C-termini are labelled with C', the N-terminal redox centre with C59/C63, and the intra-molecular disulphide between U498C′hTrxR1and C32hTrx1with disulphide. Figure 4: Close-up view of the hTrxR1-hTrx1 interface. One hTrxR1 subunit is shown in light grey, the other in dark grey and the hTrx1 molecule in blue; the C-terminal arm of the complex structure is shown in green. The conformation of the C-terminal arm and of residue E122 as found in the 'reduced waiting position' are superimposed and are coloured orange. C-termini are labelled with C', the N-terminal redox centre with C59/C63, and the intra-molecular disulphide between U498C′ hTrxR1 and C32 hTrx1 with disulphide. 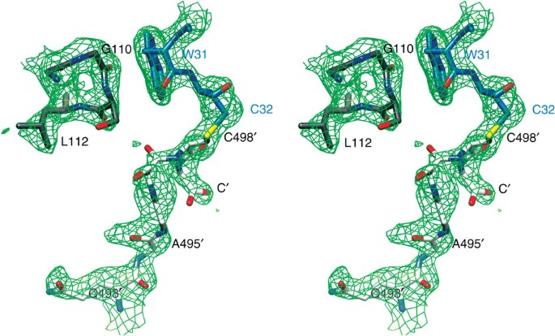Figure 5: Stereo view of a composite SA omit map. A composite SA omit map at 2.2 Å resolution and contoured at 1σ, covering a major part of the interface region of the hTrxR1–hTrx1 complex (hTrxR1, residues labelled in black; hTrx1, residues labelled in blue). Full size image Figure 5: Stereo view of a composite SA omit map. A composite SA omit map at 2.2 Å resolution and contoured at 1σ, covering a major part of the interface region of the hTrxR1–hTrx1 complex (hTrxR1, residues labelled in black; hTrx1, residues labelled in blue). Full size image Another interaction region in the complex involves several oppositely charged residues: Lys36 hTrx1 –Glu103 hTrxR1 , Asp60 hTrx1 –Arg117 hTrxR1 , Asp64 hTrx1 –Lys146 hTrxR1 , Glu70 hTrx1 –Arg121 hTrxR1 , and Lys72 hTrx1 –Glu122 hTrxR1 . Most of these residues are found in different conformations and interact through van der Waals forces, salt bridges, or hydrogen bonds. A third interaction region involves a set of inter- and intra-molecular, antiparallel β-bridges formed between hTrxR1 residues 495′ hTrxR1 to 499′ hTrxR1 and hTrx1 residues 72 hTrx1 to 75 hTrx1 ( Fig. 6 ). The active site residue C497S′ hTrxR1 is sandwiched between Ser415′ hTrxR1 and Ser111 hTrxR1 , the latter being in hydrogen bond distance (3.6 Å) to His108 hTrxR1 ( Fig. 6 ). The C-terminal region of hTrxR1 is further stabilized by the interaction of residues 494′ hTrxR1 and 495′ hTrxR1 with the previously defined 'guiding bar' Asn418′ hTrxR1 and Asn419′ hTrxR1 (ref. 16 ). All residues involved in forming the intermediate are highly conserved in mammals. 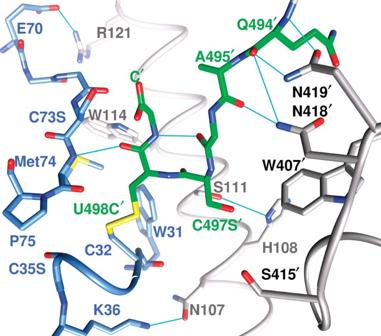Figure 6: Close-up view of the intermolecular disulphide bond. Inter- and intra-molecular, antiparallel β-bridges between hTrxR1 residues (grey, green) and hTrx1 residues (blue) and the mixed disulphide between U498C′hTrxR1and Cys32hTrx1are shown. Figure 6: Close-up view of the intermolecular disulphide bond. Inter- and intra-molecular, antiparallel β-bridges between hTrxR1 residues (grey, green) and hTrx1 residues (blue) and the mixed disulphide between U498C′ hTrxR1 and Cys32 hTrx1 are shown. Full size image Structural comparison The four independent hTrxR1 structures determined in the two crystal forms are essentially identical within the coordinate error (0.2 Å for 490 Cα-atoms). Minor variability occurs in the interface region. The first 9 N-terminal residues are not always seen in the electron density and have been omitted from the comparisons. For the substrate hTrx1, a slightly higher structural variation is observed due to the slightly more flexible region 58 hTrx1 to 74 hTrx1 (0.6 Å for 105 Cα-atoms). A comparison of hTrxR1 dimers as seen in our complex structures with published TrxR1 structures [10] , [13] , [15] , [16] (Debreczeni JE et al ., unpublished result. PDB code 2cfy) reveals a typical r.m.s. of 0.5 Å. About 965 to 976 equivalent residues were automatically determined. Non-equivalent or non-existing residues were identified near the N- and C-terminal regions. Superimposition of the hTrx1 structures obtained in the hTrxR1–hTrx1 complexes with published structures in the uncomplexed form (PDB codes 2hsh [18] , and 1aiu [17] ) also shows r.m.s. deviations of around 0.6 Å. A comparison to the hybrid enzyme TGR reveals a slightly higher r.m.s. of 0.9 Å (PDB code 2x8c) [19] . Apparently, complex formation does not induce major conformational changes in hTrxR1 or hTrx1. Structural changes seen in the complex are confined to the flexible C-terminal arm of hTrxR1. In our previously published structure of hTrxR1, we showed different distinct conformations of the C-terminal arm [16] . In one conformation, the so-called 'reduced waiting position', Cys497′ hTrxR1 and Cys498′ hTrxR1 are reduced, but the sulphur atoms are still oriented towards the inter-subunit cleft ( Fig. 4 ; PDB code 2j3n (ref. 16 ), chain C, residues: 495′ hTrxR1 to 499′ hTrxR1 ). The negative charge at the C-terminus opposes Glu122 hTrxR1 , which forms a barrier so that the mobile arm is prevented from leaving the interior of the TrxR molecule before a substrate is bound ( Fig. 4 ). A comparison to this previously published structure of hTrxR1 shows that upon binding oxidized hTrx1s, as seen in the complex structure, the side chain of Glu122 hTrxR1 rearranges. In one copy of our four complexes, Glu122 hTrxR1 interacts with Lys72 hTrx1 ; in others it points towards the solvent. Upon formation of the complex, the course of the C-terminal arm moves from its 'reduced waiting position' to the surface of hTrxR1. Its motion involves a rotation of residues 494′ hTrxR1 to 496′ hTrxR1 , which are still in contact with the guiding bar, and the last three residues 497′ hTrxR1 to 499′ hTrxR1 flip to the surface so that after rearrangement residues 495′ hTrxR1 to 499′ hTrxR1 form a beta turn ( Figs 3 , 4 , 5 ). In this structure, the C-terminal redox centre is found at least 20 Å away from the N-terminal redox centre. In the structure of the 'reduced waiting position' as well as in other structures with a reduced C-terminal active site (TGR, PDB code 2×8c (ref. 19 ); rTrxR, PDB code 3ean (ref. 15 )) the distance between the redox centres is about 13 Å ( Fig. 3 ). Furthermore, in all of these structures the C-terminal arm is aligned by the conserved guiding bar residue Asn419′ hTrxR1 (Asn518 in TGR) through a strong hydrogen bond. Functional characterization of hTrxR1 variants In order to study the impact of the guiding bar residues (Trp407′ hTrxR1 , Asn418′ hTrxR1 , and Asn419′ hTrxR1 ) of hTrxR1 upon catalysis, we constructed two different mutants of hTrxR1: hTrxR1 N419A,U498C , and hTrxR1 W407A,N418/9A,U498C ( Table 2 ). Our crystal structures suggest that the guiding bar suppresses random motions of the flexible C-terminal arm of TrxR during catalysis [16] . A disruption of the guiding bar might therefore lead to a higher flexibility of the C-terminal arm. In fact, mutational disruption of the guiding bar did leave to a clear increase in hTrx1- and DTNB-reduction activity of hTrxR1 ( Table 2 ). As expected, the strictly conserved Asn419′ hTrxR1 appears to be the most important residue for aligning the flexible C-terminal arm during catalysis, because a simultaneous mutation of all three guiding bar residues (Trp407′ hTrxR1 , Asn418′ hTrxR1 , and Asn419′ hTrxR1 ) led only to a minor increase in hTrx1- and DTNB-reduction activity of hTrxR1 compared to the mutation of Asn419′ hTrxR1 alone ( Table 2 ). Table 2 Steady-state kinetic constants of different hTrxR1 U498C variants. Full size table The interface residue Trp114 hTrxR1 is solvent exposed in uncomplexed hTrxR1 structures, but it is interlocked with several Trx-residues in the complex structure ( Figs 4 and 6 ). In order to investigate the importance of Trp114 hTrxR1 for Trx substrate binding, we mutated Trp114 to Ala. As expected, hTrxR1 W114A,U498C did not have detectable activity with hTrx1 C73S ( Table 2 ). Furthermore, we determined increased NADPH-oxidation with high concentrations of hTrxR1 W114A,U498C in the presence and absence of hTrx1 C73S in the assay ( Table 2 ). Our results are in accordance with the previously described findings that TrxR1 shows an enhanced NADPH oxidation if there is no electron transport to the substrate [20] , [21] . Our notion was further supported by the fact that with DTNB, a small artificial disulphide substrate [22] , hTrxR1 W114A,U498C showed the same kinetic constants as hTrxR1 U498C , because Trp114 hTrxR1 is not involved in binding of DTNB to the C-terminal active site ( Table 2 ). This is the first time the complex of a large, eukaryotic thioredoxin reductase, with its physiological substrate thioredoxin, has been described. We used mutants of hTrxR1 (hTrxR1 C497S,U498C ) and hTrx1 (hTrx1 C35S,C73S ) to obtain a stable hTrxR1–hTrx1 complex. The crystal structures of the complex provide new insight into the electron transport from NADPH to the oxidizing substrate mediated by the enzyme. On the basis of our data, the structures mimic the intermediate state of the mixed disulphide between TrxR and oxidized Trx as delineated below. In our structures of the hTrxR1–hTrx1 complex, the last six C-terminal residues of hTrxR1, including the second redox centre, adopt a well-defined position, and the last four residues are located at the surface of the enzyme ( Fig. 3 ). The C-terminal residues form a set of inter- and intra-molecular, antiparallel β-bridges between hTrxR1 residues 495′ hTrxR1 to 499′ hTrxR1 and hTrx1 residues 72 hTrx1 to 75 hTrx1 as well as a mixed disulphide between U498C′ hTrxR1 and Cys32 hTrx1 ( Fig. 6 ). It has been postulated before that either residue Sec498′ hTrxR1 or residue Cys497′ hTrxR1 attacks the intra-molecular hTrx1-disulphide (Cys32 hTrx1 , Cys35 hTrx1 ), forming an inter-molecular disulphide bond between hTrx1 and hTrxR1 during catalysis [23] . After deprotonation of the other, non-attacking Sec/Cys residue the mixed disulphide is resolved, resulting in the release of reduced hTrx1. The presence of the mixed disulphide observed in all of our crystallographically independent copies of the complex supports the notion that Sec498′ hTrxR1 is the attacking residue of the intra-molecular disulphide in oxidized hTrx1. Consequently Cys497′ hTrxR1 must cleave the inter-molecular disulphide. Moreover, only the mutant combinations hTrxR1 C497S,U498C and hTrx1 C35S,C73S yielded a stable complex, indicating that C32 hTrx1 is initially attacked by Sec498′ hTrxR1 of the enzyme. Interestingly, there is no His/Glu dyad in the vicinity that could be used for the deprotonation essentially involved in resolving a disulphide bond. Instead, Cys497′ hTrxR1 is sandwiched between Ser415′ hTrxR1 and Ser111 hTrxR1 , the latter being within hydrogen bond distance (3.6 Å) to a strictly conserved His108 hTrxR1 ( Fig. 6 ). This structural environment suggests that Cys497′ hTrxR1 could be deprotonated by a Ser111/His108 hTrxR1 dyad. To test this hypothesis, we generated four different hTrxR1 mutants: hTrxR1 H108L,U498C , hTrxR1 S111A,U498C , hTrxR1 S415A,U498C , and hTrxR1 H108L,S111A,U498C . Surprisingly, all mutants showed > 90% thioredoxin reducing activity in direct comparison to hTrxR1 U498C (data not shown). This renders the hypothesis of a Ser111/His108 hTrxR1 dyad for deprotonation of Cys497′ hTrxR1 unlikely. Cheng et al . [15] proposed that deprotonation of Cys497′ TrxR occurs either through direct proton transfer from Cys497′ TrxR to Cys35 Trx or via solvent water molecules. In our structure Cys497′ hTrxR1 and Cys35 hTrx1 are 10 Å apart; this distance is incompatible with a direct proton transfer between these cysteines. Our results, therefore, strongly support the hypothesis that the proton transfer from Cys497′ TrxR to Cys35 Trx occurs via solvent water molecules. The C-terminal redox centre of hTrxR1, located on a flexible arm, has been expected to act as an electron shuttle between the buried N-terminal dithiol and the substrate [16] , [24] . In our structure of the hTrxR1–hTrx1 complex, the buried dithiol is about 20 Å apart from the C-terminal active site. In uncomplexed structures of human (monE, monC, PDB code 2j3n) [16] and rat TrxR1 (PDB code 3eao and 3ean) [15] , this distance decreases to about 13 Å, implying that the flexible C-terminal arm adopts different conformations upon catalysis ( Figs 3 and 4 ). One of these conformations could be described as an 'oxidized waiting position' with an oxidized C-terminal active site (monE, PDB code 2j3n [16] , 3eao [15] ) 13 Å apart from the buried disulphide. Upon reduction of the N-terminal active site by NADPH, the C-terminal active site probably turns to the N-terminal dithiol and becomes reduced. We assume that after binding the next NADPH molecule, the re-reduced N-terminal active site repels the reduced C-terminal active site. This confirmation could be described as 'reduced waiting position' (also 13 Å apart from the N-terminal active site) with both side-chain sulphur atoms directed toward the inter-subunit cleft, making an electron transport to the substrate impossible (monC, PDB code 2j3n) [16] . Upon binding the substrate Trx, the C-terminal arm most likely turns to the surface and reduces Trx (20 Å apart, Figs 3 and 4 ). We assume that the oxidized C-terminal redox centre swings back to the conformation seen in the uncomplexed structures of TrxR1, thereby adopting the mentioned 'oxidized waiting position' again, completing the possible reaction cycle. In all conformations, the C-terminal arm forms variable hydrogen bonds to the guiding bar residues (Trp407′ hTrxR1 , Asn418′ hTrxR1 , Asn419′ hTrxR1 ). Furthermore, the hydrogen bond, which involves the conserved residue Asn419′ hTrxR1 , is also present in structures of rat TrxR and TGR with a reduced C-terminal end. Our hypothesis is strongly supported by kinetic evidence, which we gained by disrupting the residues of the guiding bar ( Table 2 ). Correspondingly, disruption of the guiding bar led to 55% and 72% increases in the catalytic efficiency of hTrxR1 for hTrx1 and for DTNB, respectively ( Table 2 ). Mutation of the strictly conserved guiding bar residue Asn419′ hTrxR1 alone led to a strong effect ( Table 2 ), rendering it the most important residue for aligning the flexible C-terminal arm during catalysis. Simultaneous mutation of all three guiding bar residues (Trp407′ hTrxR1 , Asn418′ hTrxR1 , and Asn419′ hTrxR1 ) only led to a minor increase in catalytic efficiency of hTrxR1 compared to the Asn419′ hTrxR1 mutation ( Table 2 ). The increase in catalytic efficiency can be explained by the fact that the flexible C-terminal arm is aligned by the guiding bar residues. If these contacts are disrupted through mutations in these residues, the random motions of the C-terminal arm should increase. Consequently, this leads to a faster reduction of its substrates but may also lead to an unspecific loss of electrons. Our view of the reaction cycle is also in accordance with a number of other biochemical and structural observations. It has been noted that Trxs as well as TrxRs contain solvent-exposed tryptophan residues, which are highly unfavourable energetically. Owing to complex formation, solvent-exposed Trp31 hTrx1 and Trp114 hTrxR1 fit into hydrophobic pockets in the interface region; additionally, their indole rings are in van der Waals contact. The importance of Trp114 hTrxR1 for hTrx1 binding could be supported through kinetic analysis of a hTrxR1 W114A,U498C mutant, which did not produce a detectable activity in the Trx-assay ( Table 2 ). Trp114 hTrxR1 interacts with Trp31 hTrx1 and other Trx-residues, but it is not involved in binding the small, artificial disulphide substrate DTNB [22] . Hence, if we used DTNB as substrate, the hTrxR1 W114A,U498C mutation did not influence steady-state kinetic constants compared to the hTrxR1 U498C variant ( Table 2 ). To conclude, we could provide strong evidence that Trp114 hTrxR1 is involved in hTrx1 binding, but not in the catalytic reduction mechanism itself. In previous reports, Asp60 hTrx1 has been mentioned as an important residue that quenches Trp31 hTrx1 (refs 17 , 25 ). In our complex structure, Asp60 hTrx1 is further stabilized by forming a salt bridge to Arg117 hTrxR1 ( Fig. 4 ) underlining the role of these residues for Trx binding and catalysis. In this work we used a C73S hTrx1 mutant in order to avoid formation of hTrx1 dimers involving a disulphide between Cys73 hTrx1 and C73′ hTrx1 of a second hTrx1 molecule [26] , [27] . Such Trx1-dimers are known not to be a substrate of TrxR1 (ref. 26 ). This finding can be explained by our structure, because in the presence of a disulphide between Cys73 hTrx1 and Cys73′ hTrx1 , the hTrx1 residues 73 hTrx1 to 75 hTrx1 , which are involved in binding of hTrx1 to hTrxR1 (see above), are not available for hTrxR1–hTrx1 complex formation ( Fig. 6 ). Moreover our structure is likely to explain the considerable drop in hTrx1 activities upon disulphide formation between residues Cys62 hTrx1 and Cys69 hTrx1 (ref. 28 ). Both cysteines belong to the interface region 58 hTrx1 to 74 hTrx1 and are located on the same helix separated by two turns; therefore, disulphide formation distorts the alignment of hTrx1 with hTrxR1. Other residues of the interface region in our structure have also been reported to be of importance. Pro75 hTrx1 has been shown to prevent metal binding by the reactive thiolate-based active site [29] , and residues Glu70 hTrx1 and Lys72 hTrx1 are required for procaspase-3 affinity [30] . Lys36 hTrx1 faces Glu103 hTrxR1 and is probably also involved in the docking and release of hTrx1 (ref. 31 ) ( Fig. 4 ). One region in the complex interface involves several oppositely charged residues, indicating their importance for docking and releasing hTrx1. All of the residues involved in forming the complex are strictly conserved in mammals, subsequently underlining their essential role in catalysis. The broad functional spectrum of TrxR1, its involvement in a magnitude of cellular processes, and therefore, its importance in a variety of diseases make it a highly interesting candidate for drug development [7] . To simultaneously decrease DNA synthesis and antioxidant defence of a tumour cell by the inactivation of one enzyme is indeed a tempting approach. A number of clinically and experimentally utilized chemotherapeutic drugs, including the cytostatic agent BCNU, gold and platinum complexes, and compounds acting at the dimer-interface have already been shown to inhibit TrxR1 effectively [2] , [3] , [7] . Chemotherapeutic treatment can be successfully realized by redox targeting, that is, inhibition of TrxR or Trx, in different forms of human cancer such as glioblastoma, colon, and lung and breast cancer. Moreover, it has been shown that Trx and TrxR have major roles in the denitrosylation processes controlling apoptosis [32] . Here we have described the structural characteristics of hTrxR1–hTrx1 complex formation. Complex formation does not induce gross conformational changes in TrxR or Trx. Instead, the enzyme uses a flexible C-terminal arm, which adopts different conformations during catalysis to reduce its substrates. The function of the guiding bar, as postulated in our previous report [16] , could be strengthened by the crystal structure, and disruption of the guiding bar led to an increase in Trx-reduction efficiency, which further supports its importance for regulatory processes in catalysis of TrxR1. We believe that the three-dimensional structure of the hTrxR1–hTrx1 complex will facilitate future drug discovery approaches and will significantly contribute to our understanding of redox regulatory processes in mammals. Cloning and purification Three hTrxR1 constructs were cloned into the pET28a(+) expression vector (Novagen) using Nde I and Hin dIII restriction sites: a double hTrxR1 mutant where Cys497 and Sec498 were replaced by Ser and Cys, respectively (hTrxR1 C497S,U498C ), as well as a hTrxR1 mutant where Sec498 was replaced by Ser (hTrxR1 U498S ), and a truncated form of hTrxR1 where a stop codon was introduced after Cys497 (hTrxR1 C497_trunc ). The constructs were amplified from the previously described hTrxR1 U498C construct, using OhTrxRf (5′-TATTACATATGAACGGCCCTGAAGATCTTCCCAAGTCC-3′) as forward primer, and OhTrxRrSC (5′-TATTAAAGCTTTTAACCACAGGAGCCAGCCTGGAGGAT-3′), OhTrxRrCS (5′-TATTAAAGCTTTTAACCAGAGCAGCCAGCCTGGAGGAT-3′), or OhTrxRrCtrunc (5′-TATTAAAGCTTTTAACCTTAGCAGCCAGCCTGGAGGAT-3′) as reverse primers for PCR, respectively [33] . In the two full-length constructs Sec was mutated either to Cys or Ser to enable high-yield heterologous overexpression in E. coli . The other mutation (C497S) and the truncation as well as the mentioned mutation of U498S were introduced to obtain stable protein complexes for crystallization. Recombinant, His-tagged hTrxR1 mutant proteins were overexpressed in E. coli using the pET28a(+)/BL21 Rosetta (DE3) pLysS expression system and purified by Ni-NTA affinity chromatography as described before [33] . Additionally, three hTrx1 mutants were used: hTrx1 C73S , hTrx1 C32S,C73S , and hTrx1 C35S,C73S . hTrx1 C73S and hTrx1 C32S,C73S were prepared as reported previously [34] . Mutation of Cys35 to Ser was introduced into Trx1 C73S by PCR with Pfu polymerase (Promega) using mutational primers (hTrxC35Sfor: 5′-CGTGGTGTGGGCCTTCCAAAATGATCAAGC-3′; hTrxC35Srev: 5′-GCTTGATCATTTTGGAAGGCCCACACCACG-3′). The recombinant proteins were overexpressed using the pQE30/ E. coli M15 expression system and purified by Ni-NTA affinity chromatography. The C73S mutation was present in all hTrx1 species to prevent undesirable dimer formation [26] , [27] . Complex formation and gel filtration chromatography hTrxR1 mutant proteins were incubated with a 20-molar excess of hTrx1 mutant proteins in Tris buffer (50 mM Tris-HCl, 200 mM NaCl, 1 mM EDTA, pH 7.6) containing 2.5 mM NADPH for 5 h at room temperature. After incubation, the protein solution was analysed by gel filtration chromatography on a HiLoad 16/60 Superdex 200 prep grade column (GE Healthcare), which was connected to an ÄKTA–FPLC system (GE Healthcare). FPLC fractions were detected spectrophotometrically, and peak areas and k AV -values were evaluated using the software UNICORN 4.11 (GE Healthcare). Protein complex containing FPLC fractions were analysed by non-reducing 10% SDS-polyacrylamide gel electrophoresis (SDS–PAGE). Crystallization Mutants (see above) of hTrxR1, complexed with hTrx1 in 50 mM Tris-HCl, 200 mM NaCl, 1 mM EDTA, pH 7.6, were concentrated to 10 mg ml −1 . Crystals were grown at 24 °C in hanging drops by the vapour diffusion technique. The reservoir of the monoclinic crystals contained 15% PEG 4000, and the reservoir of orthorhombic crystals contained 15% PEG 6000, MES 0.1 M, pH 6.5. Before the measurements, the crystals were soaked in mother liquour containing a final concentration of 20% glycerol. Data collection All diffraction data were recorded by the rotation method and processed with XDS [35] . We obtained monoclinic (space group P2 1 ) and orthorhombic crystals (space group P2 1 2 1 2 1 ) of hTrxR1 C497S,U498C in complex with its substrate hTrx1 C35S,C73S . The crystals of both types contained two copies of the hTrxR1–hTrx1 complex in the asymmetric unit thereby maintaining the usual hTrxR1 dimer. A complete monoclinic dataset to 2.6 Å resolution and, owing to radiation damage, a less complete orthorhombic dataset to 2.2 Å resolution ( Table 1 ) were collected at 100°K using synchrotron radiation (SLS, Paul Scherrer Institute, Villigen, Suisse, beamline X10SA; rotation/image: 1.0°, λ=1 Å (monoclinic); rotation/image: 1.0°, λ=1.0068 Å (orthorhombic), detector CCD, (MARCCD)). Structure determination Reflection phasing and structure refinements were carried out using the cns program suite [36] . Structure solution was started with the monoclinic crystal data (which were available first) using the molecular replacement method. The starting model consisted of the human TrxR1 dimer (PDB code 2j3n) [16] without the 10 N-terminal and 20 C-terminal TrxR residues known to be flexible. The automatic program packages [36] , [37] identified the correct positions of the hTrxR1 dimer. The search model was augmented subsequently by the small hTrx1 (PDB code 1aiu) [17] molecules but the programs failed to reveal their correct position, presumably because of the intricate packing of the molecules in the crystal. However, the 2Fo-Fc map showed regions of helical density that served as an anchor point to position manually one hTrx1 molecule using the interactive graphics program O (ref. 38 ). The second hTrx1 molecule was generated by application of the twofold rotation of the TrxR dimer, and subsequent rigid-body refinement. This model (without the last C-terminal residues) was used as a starting model for the orthorhombic crystal form. Refinement was completed after several rounds of model correction, thereby imposing non-crystallographic restraints on residues 15:50, 54:81, 100:106, 135:220, 227:240, 279:335, 342:410, 412:428, and 434:490. Structure assignment of the C-terminal loop was initially based on the best interpretable density region of the two complexes of the orthorhombic crystal forms. After refinement, annealed omit maps were used to correct the course of the C-terminal chain residues in both orthorhombic and monoclinic crystal forms ( Fig. 5 ). The models show good stereo-chemistry ( Table 1 ) as verified by procheck [39] . Coordinates and measured reflection amplitudes were deposited in the Brookhaven Protein Data Bank (PDB code 3QFA, and 3QFB). Construction of further hTrxR1 variants On the basis of the information provided by the crystal structure of the complex, 3 hTrxR1 mutants were produced from the hTrxR1 U498C mutant described above (hTrxR1 W114A,U498C , hTrxR1 N419A,U498C , and hTrxR1 W407A,N418/9A,U498C ). Mutations were inserted through site-directed mutagenesis using the Quick Change II Site Directed Mutagenesis Kit (Stratagene). Following primers were used to generate the W114A mutation: forward 5′-GCTCTTTGAATTCGGGCTACCGAGTAG-3′ and reverse 5′-CTACTCGGTAGCCCGAATTCAAAGAGC-3′, as well as forward 5′-GCTCTTTGAATGCGGGCTACCGAGTAG-3′ and reverse 5′-CTACTCGGTAGCCCGCATTCAAAGAGC-3′. Following primers were used to generate the N419A mutation: forward 5′-CCGTCAAGAGATAACGCCAAATGTTATGCAA-3′ and reverse 5′-TTGCATAACATTTGGCGTTATCTCTTGACGG-3′. Following primers were used to generate the N418/9A mutation: forward 5′-GAATGGACGATTCCGTCAAGAGATGCCGCCAAATGTTATGCAA-3′ and reverse 5′-TTGCATAACATTTGGCGGCATCTCTTGACGGAATCGTCCATTC-3′. Following primers were used to generate the W407A mutation: forward 5′-CCATAGTTACTTTTCGCCATTGGAATGGAC-3′ and reverse 5′-GTCCATTCCAATGGCGAAAAGTAACTATGG-3′, as well as forward 5′-CCATAGTTACTTTGCGCCATTGGAATGGAC-3′ and reverse 5′-GTCCATTCCAATGGCGCAAAGTAACTATGG-3′. After sequencing, the correct plasmids were transformed into E. coli BL21 Rosetta (DE3) cells and expressed and purified as described above. Kinetic characterization of hTrxR1 variants The data for the enzyme kinetics were obtained using a U-2100 UV/Vis spectrophotometer (Hitachi). hTrxR1 activity was measured using 5,5′-dithiobis(2-nitrobenzoic acid) (DTNB) [22] as well as a hTrx1 mutant (C73S) [34] as substrates. The NADPH-dependent reduction of DTNB/hTrx1 in 100 mM phosphate buffer, 1 mM EDTA, pH 7.4 was determined as the increase/decrease in absorbance at 412 nm/340 nm at 25°C (ɛ412 nm=13.6 mM −1 cm −1 ; ɛ340 nm=6.22 mM −1 cm −1 ). For each data point, the initial velocity was determined at least in triplicate over at least 12 different substrate concentrations in 3 independent experiments. Control assays lacking the substrate were routinely included as references. Accession codes: Coordinates and structure factors were deposited in Protein Data Bank with the accession codes 3QFA (orthorhombic crystals) and 3QFB (monoclinic crystals). How to cite this article: Fritz-Wolf, K. et al . Crystal structure of the human thioredoxin reductase–thioredoxin complex. Nat. Commun. 2:383 doi: 10.1038/ncomms1382 (2011).